The ancestral role of nodal signalling in breaking L/R symmetry in the vertebrate forebrain Left-right asymmetries in the epithalamic region of the brain are widespread across vertebrates, but their magnitude and laterality varies among species. Whether these differences reflect independent origins of forebrain asymmetries or taxa-specific diversifications of an ancient vertebrate feature remains unknown. Here we show that the catshark Scyliorhinus canicula and the lampreys Petromyzon marinus and Lampetra planeri exhibit conserved molecular asymmetries between the left and right developing habenulae. Long-term pharmacological treatments in these species show that nodal signalling is essential to their generation, rather than their directionality as in teleosts. Moreover, in contrast to zebrafish, habenular left-right differences are observed in the absence of overt asymmetry of the adjacent pineal field. These data support an ancient origin of epithalamic asymmetry, and suggest that a nodal-dependent asymmetry programme operated in the forebrain of ancestral vertebrates before evolving into a variable trait in bony fish. The vertebrate epithalamus derives from a highly conserved diencephalic subdivision, which gives rise to two distinct moieties, the bilaterally paired habenular nuclei and the pineal complex. The latter comprises the pineal organ, present in all vertebrates, and a more variable structure referred to as the parapineal organ, present in teleosts and cyclostomes. The habenulae belong to an ancient conduction system connecting the limbic forebrain to the brainstem and are known to control monoaminergic activity levels in the central nervous system. They have recently aroused a renewed interest as key regulators of adaptive behaviours such as experience-dependent fear responses [1] , [2] , [3] . A remarkable property of habenulae is that they exhibit marked left-right asymmetries in size, gene expression and neuronal organization in a number of species belonging to all major vertebrate taxa [3] , [4] , [5] , albeit with a high degree of variability in asymmetry magnitude and laterality [4] , [6] . In the zebrafish, these neuroanatomical asymmetries correlate with markedly different habenulae responses to sensory stimuli [7] , [8] . Habenular asymmetry thus provides a model system to (i) decipher the mechanisms underlying L/R asymmetry diversification in vertebrates and (ii) study the relationship between behavioural and morphological adaptations related to forebrain asymmetries throughout vertebrate evolution. How the mechanisms controlling the development of habenular asymmetries have evolved across vertebrates is largely unknown. Extensive work on the ontogeny of habenular asymmetry in zebrafish has revealed that distinct developmental programmes control the generation of asymmetry per se and its directionality (reviewed in refs 3 , 4 , 5 , 9 ). In this species, a left-handed expression of nodal pathway components and downstream target Pitx2 is the first molecular indication of a diencephalic asymmetry. The role of nodal is to control asymmetry laterality rather than its establishment per se , as abrogation of nodal signalling results in the randomization of habenular asymmetry rather than its total loss [10] , [11] . In addition, Fgf8-dependent lateralized migration of the parapineal rudiment plays a key part in the establishment of proper habenular asymmetries, as shown by the right isomerism phenotype observed following parapineal laser ablation or in zebrafish mutants exhibiting parapineal migration or specification defects [12] , [13] , [14] . Whether these mechanisms have been conserved throughout vertebrate evolution remains unclear. Asymmetric nodal expression in the forebrain, for instance, has only been reported in teleosts [10] , [15] , [16] . Analyses of habenular asymmetry establishment in agnathans (or cyclostomes) and cartilaginous fishes (or chondrichthyans) are of major interest to address this issue. Indeed, as, respectively, sister groups of gnathostomes (or jawed vertebrates) and osteichthyans (that is, the third main vertebrate lineage including bony fishes and tetrapods), they occupy key phylogenetic positions to decipher vertebrate ancestral mechanisms and unravel the evolution of asymmetry diversification in different vertebrate lineages [17] . Although both agnathans and chondrichthyans exhibit marked asymmetries in size and neuronal organization between the left and right habenulae [4] , [18] , [19] , [20] , [21] , the existence of conserved pineal-dependent habenular asymmetry as in zebrafish remains unclear in these taxa. Indeed, contrary to the zebrafish, habenular asymmetry establishment in lampreys (cyclostomes) precedes parapineal segregation from the pineal anlage [18] , [22] , [23] , [24] , [25] , [26] . Furthermore, the parapineal organ does not migrate to the left as it does in the zebrafish epithalamus but remains at the midline. Finally parapineal axon projections to the left habenula [22] occur at larval stages, that is, well after the habenulae have acquired their L/R identity. Along the same line, chondrichthyans have been reported to lack a parapineal organ and neither neurochemical descriptions nor tract-tracing analyses have been able to reveal asymmetric pineal projections [6] , [27] , [28] . Here, we address the origin and evolution of vertebrate epithalamic L/R asymmetries by analysing the mechanisms controlling their formation in two lamprey species ( Petromyzon marinus and Lampetra planeri ) and in the catshark ( Scyliorhinus canicula) , representatives of cyclostomes and chondrichthyans, respectively. We investigate the role of nodal in setting up habenular L/R asymmetry in both species. We show that, although habenular molecular asymmetries are conserved in cyclostomes, chondrichthyans and teleosts, habenular asymmetry in the catshark and lampreys occurs in a nodal-dependent manner, with nodal playing a pivotal role in the generation of L/R asymmetry per se . Our work thus highlights an ancient genetic programme already operating in the last common ancestor of vertebrates, and provides an entry point to explore the link between epithalamic asymmetry diversification and behavioural adaptation in the major vertebrate lineages. Conserved diencephalic molecular asymmetries in vertebrates Orthologues of Nodal , Lefty and Pitx2 , three key components of the nodal pathway, can be identified in the catshark and lamprey ( Fig. 1 , phylogenetic analyses in Supplementary Fig. 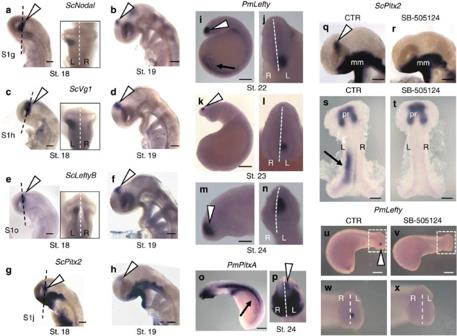Figure 1: ANodal-Lefty-Pitxcassette is asymmetrically expressed in the diencephalon of catshark and lamprey embryos. (a–h)ScNodal,ScVg1,ScLeftyBandScPitx2expression in the catshark. (a–h) Represent left lateral views of catshark embryos after hybridization withScNodal(a,b),ScVg1(c,d),ScLeftyB(e,f) andScPitx2(g,h) probes. (a,c,e,g) and (b,d,f,h) show stage 18 and 19 embryos, respectively. Insets show dorsal views of the head region of the embryos shown in (a,c,e), confirming the left-restricted diencephalic expression of each gene. (i–p)PmLeftyandPmPitxAexpression in the lampreyP. marinus. (i,k,m,o) Represent left lateral views of lamprey embryos from stage 22 to stage 24 as indicated after hybridization withPmLefty(i–m) andPmPitxA(o) probes. Higher magnification of the head region inm. Frontal views of the head region of the embryos (i,k,m,o) are shown in (j,l,n,p), confirming the left-restricted diencephalic expression ofLeftyandPitxA. (q–x) Effect of SB-505124 treatment onScPitx2andPmLeftyexpression. (q–t) Show the expression pattern ofScPitx2in catshark embryos following short-term treatment with DMSO (CTR:q,s) or with a nodal/activin inhibitor (SB-505124:r,t). (q,r) Show left lateral views of the head region, (s,t) dorsal views. Treatments were conducted from stage 13 to 14 (s,t) or from stage 15 to 16 (q,r), respectively, resulting in the loss of LPM or diencephalonScPitx2expression. Similar results were obtained using a lower dose (50 μM) of SB-505124 (Supplementary Table 3). (u,v) Show the expression pattern ofPmLeftyin lamprey (L. planeri) embryos treated with DMSO (CTR:u) or with a nodal/activin inhibitor SB-505124 (v). (w,x) Higher magnification of the boxed areas in (u,v), showing front views of the head region. Dotted black lines indicate planes of the sections shown inSupplementary Fig. 1g–j. Dotted white lines mark the location of the midline. Black arrows and white arrowheads, respectively, point to gene expressions in the left LPM and in the diencephalon. L=left; mm=mandibular mesoderm; pr=pharyngeal region; R=right. Scale bars, 200 μm, except inm, 100 μM. 1a ; Supplementary Table 1 ). As described in the zebrafish, the catshark orthologues of Nodal , Vg1 , Lefty and Pitx2 ( ScNoda l, ScVg1 , ScLeftyB and ScPitx2 ) and lamprey P. marinus orthologues PmPitxA and PmLefty are expressed in the left part of the lateral plate mesoderm (LPM) at neural plate stages ( Supplementary Fig. 1b–f ; Fig. 1i,l ). Dorsal diencephalon expression in both the catshark and lamprey begins after neural tube closure, from stages 17 to 20 in the catshark and stages 22 to 24 in the lamprey. In both species, all the analysed nodal pathway components are expressed on the left side of the dorsal diencephalon ( Figs 1a–o ; Supplementary Fig. 1g–j ). In the catshark, ScPitx2 is detected throughout all stages analysed ( Fig. 1g,h ; Supplementary Fig. 2a–c , see below), while in the lamprey, PmPitxA transcripts remain undetectable except at stage 24 (see below Fig. 2 and Supplementary Fig. 2 ). 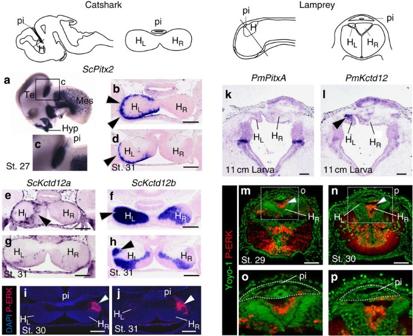Figure 2: Conserved molecular asymmetries in the developing habenulae of the catshark and lamprey. The two drawings at the top of each panel correspond to schematic representations of the embryonic catshark (left panel) and lamprey (right panel) brains showing pineal organ and habenulae location. Dotted lines indicate section planes. A schematic representation of these sections is shown beside the drawings. (a–h) Asymmetric expression ofScPitx2, ScKctd12aandScKctd12bin the catshark developing habenulae and ofPmPitxAandPmKctd12inP. marinusdeveloping habenulae (k,l). (a,c) Display left lateral views of a stage 27 catshark brain after whole-mount hybridization with aScPitx2probe, (c) corresponding to a higher magnification of the region boxed in (a). (b,d), (e,g), (f,h) Show transverse sections of stage 31 habenulae (level ofd,g,hmore posterior thanb,e,f), followingin situhybridization withScPitx2, ScKctd12aandScKctd12bprobes, respectively. Note that, at this stage, the size difference between the left and right habenulae is visible at anterior levels. (k) and (l) show habenulae transverse sections of a 11-cmP. marinuslarva, followingin situhybridization withPmPitxAandPmKctd12probes, respectively. Section planes are oriented as shown on the schemes on the top of the figure. (i,jandm–p) Differential accumulation of P-ERK in the left and right habenulae in the catshark and the lamprey. (i,j) and (m,n), respectively, show transverse sections of developing habenulae in stage 30–31 catshark embryos and in stage 29–30 lamprey prolarvae, following fluorescent immunohistochemistry using an anti P-ERK antibody. The fluorescent P-ERK signal is shown in red, nuclei were stained with DAPI (blue,i,j) or YOYO-1 (green,m–p). (o) and (p) show close-up views of the epithalamic regions boxed in (m) and (n), respectively. Black and white arrowheads point to left-sidedin situhybridization and right-sided immunohistochemistry signals in (b,d,e,f,h,l) and (i,j,m,n), respectively. HLand HR=left and right habenulae; Hyp=hypothalamus; Mes=mesencephalon; pi=pineal organ; tel=telencephalon. Scale bars: (b–j), 200 μm; (k–n), 50 μm. Importantly, asymmetric diencephalic expression of the Nodal-Lefty-Pitx cassette is observed on the left side in 100% of analysed embryos ( Supplementary Table 2 ). Figure 1: A Nodal-Lefty-Pitx cassette is asymmetrically expressed in the diencephalon of catshark and lamprey embryos. ( a – h ) ScNodal , ScVg1 , ScLeftyB and ScPitx2 expression in the catshark. ( a – h ) Represent left lateral views of catshark embryos after hybridization with ScNodal ( a , b ), ScVg1 ( c , d ), ScLeftyB ( e , f ) and ScPitx2 ( g , h ) probes. ( a , c , e , g ) and ( b , d , f , h ) show stage 18 and 19 embryos, respectively. Insets show dorsal views of the head region of the embryos shown in ( a , c , e ), confirming the left-restricted diencephalic expression of each gene. ( i – p ) PmLefty and PmPitxA expression in the lamprey P. marinus . ( i , k , m , o ) Represent left lateral views of lamprey embryos from stage 22 to stage 24 as indicated after hybridization with PmLefty ( i – m ) and PmPitxA ( o ) probes. Higher magnification of the head region in m . Frontal views of the head region of the embryos ( i , k , m , o ) are shown in ( j , l , n , p ), confirming the left-restricted diencephalic expression of Lefty and PitxA . ( q – x ) Effect of SB-505124 treatment on ScPitx2 and PmLefty expression. ( q – t ) Show the expression pattern of ScPitx2 in catshark embryos following short-term treatment with DMSO (CTR: q , s ) or with a nodal/activin inhibitor (SB-505124: r , t ). ( q , r ) Show left lateral views of the head region, ( s , t ) dorsal views. Treatments were conducted from stage 13 to 14 ( s , t ) or from stage 15 to 16 ( q , r ), respectively, resulting in the loss of LPM or diencephalon ScPitx2 expression. 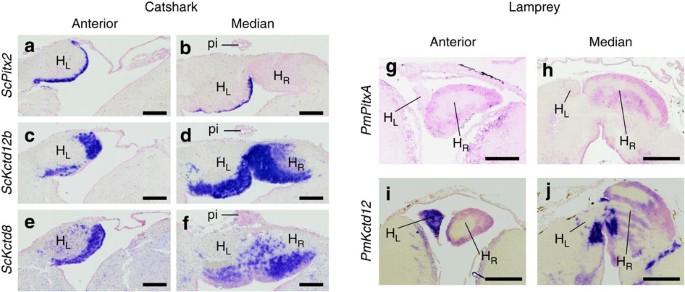Figure 3: Molecular and anatomical asymmetries are maintained in the catshark and lamprey adult habenulae. (a–f) Show transverse sections through the adult catshark habenulae at anterior (a,c,e) and median (b,d,f) levels, followingin situhybridization with the indicated probes (a,b:ScPitx2;c,d:ScKctd12b;e,f:ScKctd8). Only the left habenula appears in the anterior sections due to its larger size. The left-sided expression ofScPitx2(a,b) is maintained in the adult whileScKctd12b(c,d) andScKctd8(e,f) exhibit a bilateral albeit asymmetric expression. (g–j) Show transverse sections through the adult habenulae inP. marinusat anterior (g,i) and median (h,j) levels, followingin situhybridization with the indicated probes (g,h:PmPitxA;i,j:PmKctd12). Scale bars, 200 μm. pi=pineal stalk; HL=left habenula; HR=right habenula. Similar results were obtained using a lower dose (50 μM) of SB-505124 ( Supplementary Table 3 ). ( u , v ) Show the expression pattern of PmLefty in lamprey ( L. planeri ) embryos treated with DMSO (CTR: u ) or with a nodal/activin inhibitor SB-505124 ( v ). ( w , x ) Higher magnification of the boxed areas in ( u , v ), showing front views of the head region. Dotted black lines indicate planes of the sections shown in Supplementary Fig. 1g–j . Dotted white lines mark the location of the midline. Black arrows and white arrowheads, respectively, point to gene expressions in the left LPM and in the diencephalon. L=left; mm=mandibular mesoderm; pr=pharyngeal region; R=right. Scale bars, 200 μm, except in m , 100 μM. Full size image Figure 2: Conserved molecular asymmetries in the developing habenulae of the catshark and lamprey. The two drawings at the top of each panel correspond to schematic representations of the embryonic catshark (left panel) and lamprey (right panel) brains showing pineal organ and habenulae location. Dotted lines indicate section planes. A schematic representation of these sections is shown beside the drawings. ( a – h ) Asymmetric expression of ScPitx2, ScKctd12a and ScKctd12b in the catshark developing habenulae and of PmPitxA and PmKctd12 in P. marinus developing habenulae ( k , l ). ( a , c ) Display left lateral views of a stage 27 catshark brain after whole-mount hybridization with a ScPitx2 probe, ( c ) corresponding to a higher magnification of the region boxed in ( a ). ( b , d ), ( e , g ), ( f , h ) Show transverse sections of stage 31 habenulae (level of d , g , h more posterior than b , e , f ), following in situ hybridization with ScPitx2, ScKctd12a and ScKctd12b probes, respectively. Note that, at this stage, the size difference between the left and right habenulae is visible at anterior levels. ( k ) and ( l ) show habenulae transverse sections of a 11-cm P. marinus larva, following in situ hybridization with PmPitxA and PmKctd12 probes, respectively. Section planes are oriented as shown on the schemes on the top of the figure. ( i , j and m – p ) Differential accumulation of P-ERK in the left and right habenulae in the catshark and the lamprey. ( i , j ) and ( m , n ), respectively, show transverse sections of developing habenulae in stage 30–31 catshark embryos and in stage 29–30 lamprey prolarvae, following fluorescent immunohistochemistry using an anti P-ERK antibody. The fluorescent P-ERK signal is shown in red, nuclei were stained with DAPI (blue, i , j ) or YOYO-1 (green, m – p ). ( o ) and ( p ) show close-up views of the epithalamic regions boxed in ( m ) and ( n ), respectively. Black and white arrowheads point to left-sided in situ hybridization and right-sided immunohistochemistry signals in ( b , d , e , f , h , l ) and ( i , j , m , n ), respectively. H L and H R =left and right habenulae; Hyp=hypothalamus; Mes=mesencephalon; pi=pineal organ; tel=telencephalon. Scale bars: ( b – j ), 200 μm; ( k – n ), 50 μm. Full size image In the zebrafish, Pitx2 and Lefty are downstream targets of nodal signalling. In the catshark, nodal inhibition through pharmacological treatment using the nodal antagonist SB-505124 leads to the loss of ScPitx2 transcripts specifically in the LPM, when injections are performed at stages 13–14, that is, before nodal expression in the LPM ( Supplementary Table 3 ; compare Fig. 1s,t ). When conducted at stage 15–16, just before the start of nodal pathway activation in the central nervous system, SB-505124 injections result in specific loss of nodal activation markers in the diencephalon of both catshark and lamprey P. marinus early embryos ( Supplementary Table 3 ; compare Fig. 1q,r ; Supplementary Fig. 1k and compare Fig. 1u–x ). In contrast, catshark ScPitx2 LPM asymmetric expression, as well as its symmetric expression in the pharyngeal region or in the mandibular mesoderm, is not affected in these conditions ( Fig. 1q,r and Supplementary Fig. 1k ). Taken together, these results indicate that left-sided diencephalic expression of the Nodal-Lefty-Pitx cassette is present in the catshark and lamprey, with a robust laterality in both species. Conserved habenular asymmetries in catshark and lamprey On the basis of the relative habenulae size, larger on the left in chondrichthyans and on the right in lampreys, the directionality of epithalamic asymmetries is thought to differ between these two taxa [4] . However, such variations are not supported by the results above showing laterality conservation of the Nodal-Lefty-Pitx cassette on the left side of the diencephalon in the catshark and lamprey. Analysis of the expression of habenular asymmetric molecular markers described in teleosts allows further comparisons of the laterality of epithalamic asymmetries between both species. In the catshark, the size difference between the left and right habenulae becomes evident in the anterior-most part of the developing habenulae at stage 31 ( Supplementary Fig. 2g ). A left restricted ScPitx2 expression persists in these structures from stages 27 to 31 ( Fig. 2a–d ; Supplementary Fig. 2a–c ). As in the zebrafish [12] , [29] , expression of the catshark kctd orthologues ( ScKctd12a, ScKctd12b , ScKctd8 ) is not restricted to one side, although their expression appears stronger in the left habenula as early as stage 29 ( Supplementary Fig. 2d–f ). The asymmetry of ScKctd12a , ScKctd12b and ScKctd8 in the left and right habenulae is significantly enhanced at stage 31, with additional territories in the left habenula ( Fig. 2e–h ; Supplementary Fig. 2g ). Laterality of ScPitx2 expression is conserved in the catshark adult brain ( Fig. 3a,b ). In contrast, ScKctd8 and ScKctd12b are expressed in both left and right adult habenulae, albeit with different patterns ( Fig. 3c–f ), as previously described in zebrafish larvae [29] . In the lamprey, a marked size difference between the two habenulae is already visible in stage 27 prolarvae [30] (see below). However, the single member of the Kctd8/12/16 family, termed PmKctd12 (based on its close relationship with the Kctd12 class; Supplementary Fig. 1a and Supplementary Table 5 ), is first expressed at larval stage, restricted to the left habenulae ( Fig. 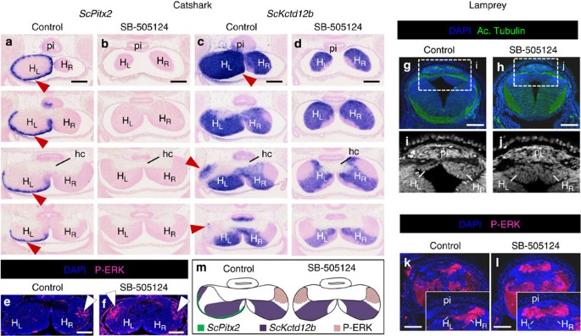Figure 5: Nodal abrogation induces a right isomerism in the catshark and lamprey epithalami. (a–f) Effect of SB-505124 treatment on habenular development in the catsharkS. canicula. (a–f) Show transverse sections of stage 31 control embryos (a,c,e) and SB-505124-treated embryos (b,d,f), following hybridization withScPitx2(a,b) andScKctd12b(c,d) probes, or following immunohistochemistry using an antibody directed against P-ERK (e,f). In (a–d), successive section planes are shown from anterior to posterior levels, with the same orientation as depicted inFig. 2. (e,f) Show sections at a median level. Red arrowheads in (a,c) point to left-sided hybridization signals present in control embryos but lost in SB-505124 treated embryos. White arrowheads in (e) point to P-ERK signals, restricted to the right in untreated or DMSO-injected embryos but found on both sides in SB-505124-treated embryos (f). A size difference is observed between the left and the right habenulae at anterior levels (larger on the left) in control embryos. Treated embryos exhibit a size reduction of the left habenula. (g–l) Effect of SB-505124 treatment on habenular development in the lampreyL. planeri. (g–l) Show transverse sections of stage 27 (g,h) and stage 30 (k,l) embryos following DAPI staining (blue) and immuno-histochemistry with an anti-acetylated tubulin (g,h; green) and an anti-P-ERK antibody (k,l; red). (i) and (j) show DAPI staining of the region boxed in (g) and (h), respectively, at higher magnification. Control embryos (g,i,k) exhibit a larger size of the right habenula and an asymmetric right P-ERK activity (k). In SB-505124-treated embryos (h,j,l), a size increase of the left habenula, resulting in a right isomerism, is observed (j) and the P-ERK signal is equally distributed between the left and right habenulae (l). Insets in (k,l) represent close-up views of the developing epithalamus. (m) Scheme showing molecular changes in habenulae of control and SB-505124-treated embryos. hc=habenular commissure; HL=left habenula; HR=right habenula; pi=pineal stalk. Scale bars: (a–f), 200 μm; (g,l), 100 μm. 2l ). In the adult, however, PmKctd12 expression is present on both sides, albeit asymmetrically as an anterior signal is only observed in the left habenula ( Fig. 3i,j ). PmPitxA expression is undetectable in the habenulae at these stages ( Figs 2k and 3g,h ). Fgf signalling plays a key role in the generation of habenular asymmetries in the zebrafish. Interestingly, analysis of MAPK-ERK activity in the catshark and lamprey epithalami highlights a strong signal exclusively in the right habenula in both species ( Fig. 2i,j,m–p ). In the catshark, P-ERK is first observed at stage 30 in the dorso-lateral part of the right habenula, and more prominently so at stage 31 ( Fig. 2i,j ; bright fields shown in Supplementary Fig. 2i,j ). This molecular asymmetry is conserved in P. marinus in which a strong P-ERK habenular signal is observed starting from stage 29, with a clear restriction on the right side ( Fig. 2m–p ). These data provide the first evidence of an asymmetric MAPK-ERK activity in the vertebrate habenulae. As was the case for the Nodal-Lefty-Pitx cassette, no evidence for a laterality shift of these molecular markers was observed in any of the embryos analysed ( n =36). Taken together, these data highlight conservations of molecular habenular asymmetries between the catshark and lamprey, with the same laterality. Figure 3: Molecular and anatomical asymmetries are maintained in the catshark and lamprey adult habenulae. ( a – f ) Show transverse sections through the adult catshark habenulae at anterior ( a , c , e ) and median ( b , d , f ) levels, following in situ hybridization with the indicated probes ( a , b : ScPitx2 ; c , d : ScKctd12b ; e , f : ScKctd8 ). Only the left habenula appears in the anterior sections due to its larger size. The left-sided expression of ScPitx2 ( a , b ) is maintained in the adult while ScKctd12b ( c , d ) and ScKctd8 ( e , f ) exhibit a bilateral albeit asymmetric expression. ( g – j ) Show transverse sections through the adult habenulae in P. marinus at anterior ( g , i ) and median ( h , j ) levels, following in situ hybridization with the indicated probes ( g , h : PmPitxA ; i , j : PmKctd12 ). Scale bars, 200 μm. pi=pineal stalk; H L =left habenula; H R =right habenula. Full size image Symmetric early pineal development in lamprey and catshark Migration of the parapineal rudiment is required for the elaboration of habenular asymmetry in zebrafish. Whether morphogenesis of the lamprey and the catshark pineal field may also be asymmetric at stages preceding, or concomitant with, the establishment of habenular asymmetries is currently unknown. In the catshark, pineal evagination above the developing habenulae begins at stage 21 (ref. 31 ) and progresses symmetrically, keeping the same proportion between the left and right sides ( Supplementary Figs 3 , 4b,c ). No asymmetric pineal cell cluster protrusion can be detected through stages 21 to 32, as assessed by the expression of pineal complex marker ScOtx5 ( Fig. 4a–d ; Supplementary Fig. 4c ), suggesting absence of pineal asymmetry or migration before the establishment of habenular L/R identity. In addition, no expression of ScGfi1 , the catshark orthologue of the zebrafish-specific parapineal marker Gfi1 (ref. 32 ) (see phylogenetic analysis in Supplementary Fig. 1a ), can be observed at the level of the pineal or habenulae ( Supplementary Fig. 4d,e ). Finally, no evidence for a diencephalic expression of ScFgf8 can be detected from stage 19 onwards ( Supplementary Fig. 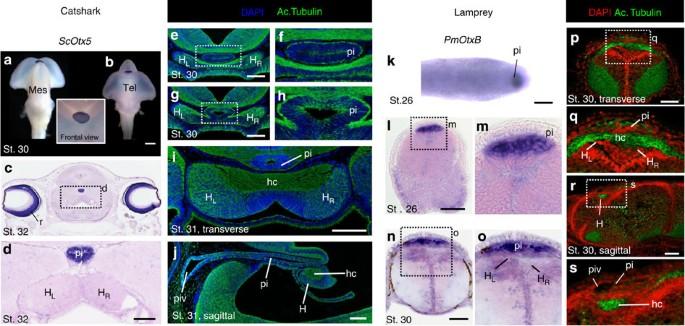4a,b ), providing evidence against conservation in the catshark of Fgf8 role in parapineal specification and migration. Figure 4: Absence of overt pineal complex asymmetry in catshark embryos or lamprey prolarvae. (a–j) Characterization of the developing pineal organ in the catshark. (a,b) Show whole-mount views of stage 30 catshark brain following hybridization with aScOtx5probe (dorsal views in (a) antero-ventral view in (b)). (c,d) Show transverse sections through the habenular region and the pineal stalk at stage 32, following hybridization with aScOtx5probe (dhigher magnification of the region boxed inc). (e–j) Show sections of the developing epithalamus in catshark embryos following immunohistochemistry with an antibody directed against acetylated tubulin (green) and DAPI staining (blue). (e,g) Represent consecutive transverse sections at the basis of the pineal stalk at stage 30. (f) and (h) are enlarged views of the region boxed in (e) and (g), respectively. (i) and (j) are, respectively, transverse and sagittal sections of the catshark epithalamus at stage 31. (k–s) characterization of the developing pineal organ in the lampreyP. marinus. (k) Shows the dorsal view of the head region of a lamprey prolarva (stage 26, anterior to the right) following whole-mount hybridization with aPmOtxBprobe. (l) and (n) show transverse sections of stage 26 and 30 lamprey prolarvae following hybridization with aPmOtxBprobe. (m) and (o) Represent close-up views of the boxed areas in (l) and (n), respectively. (p,r) Show sections of the developing epithalamus in lamprey prolarvae following immunohistochemistry with an anti-acetylated tubulin antibody (green) and DAPI staining (red, pseudocolour). (p) and (r) respectively show transverse and sagittal sections of a stage 30 prolarva, (q) and (s) represent close-up views of the areas boxed in (p) and (s). Strong staining at the base of the pineal stalk in (e,i) (catshark) and (p) (lamprey) corresponds to the habenular commissure between the left and right habenulae. This structure is also visible on sagittal sections (catshark,j; lamprey,s). H=habenulae; hc=habenular commissure; HL=left habenula; HR=right habenula; Mes=mesencephalon; pi=pineal stalk; piv=pineal vesicle; Tel=telencephalon; r=retina. Scale bars: (a), 500 μm; (d,e–j), 200 μm; (k–r), 50 μm. Figure 4: Absence of overt pineal complex asymmetry in catshark embryos or lamprey prolarvae. ( a – j ) Characterization of the developing pineal organ in the catshark. ( a , b ) Show whole-mount views of stage 30 catshark brain following hybridization with a ScOtx5 probe (dorsal views in ( a ) antero-ventral view in ( b )). ( c , d ) Show transverse sections through the habenular region and the pineal stalk at stage 32, following hybridization with a ScOtx5 probe ( d higher magnification of the region boxed in c ). ( e – j ) Show sections of the developing epithalamus in catshark embryos following immunohistochemistry with an antibody directed against acetylated tubulin (green) and DAPI staining (blue). ( e , g ) Represent consecutive transverse sections at the basis of the pineal stalk at stage 30. ( f ) and ( h ) are enlarged views of the region boxed in ( e ) and ( g ), respectively. ( i ) and ( j ) are, respectively, transverse and sagittal sections of the catshark epithalamus at stage 31. ( k – s ) characterization of the developing pineal organ in the lamprey P. marinus . ( k ) Shows the dorsal view of the head region of a lamprey prolarva (stage 26, anterior to the right) following whole-mount hybridization with a PmOtxB probe. ( l ) and ( n ) show transverse sections of stage 26 and 30 lamprey prolarvae following hybridization with a PmOtxB probe. ( m ) and ( o ) Represent close-up views of the boxed areas in ( l ) and ( n ), respectively. ( p , r ) Show sections of the developing epithalamus in lamprey prolarvae following immunohistochemistry with an anti-acetylated tubulin antibody (green) and DAPI staining (red, pseudocolour). ( p ) and ( r ) respectively show transverse and sagittal sections of a stage 30 prolarva, ( q ) and ( s ) represent close-up views of the areas boxed in ( p ) and ( s ). Strong staining at the base of the pineal stalk in ( e , i ) (catshark) and ( p ) (lamprey) corresponds to the habenular commissure between the left and right habenulae. This structure is also visible on sagittal sections (catshark, j ; lamprey, s ). H=habenulae; hc=habenular commissure; H L =left habenula; H R =right habenula; Mes=mesencephalon; pi=pineal stalk; piv=pineal vesicle; Tel=telencephalon; r=retina. Scale bars: ( a ), 500 μm; ( d , e – j ), 200 μm; ( k – r ), 50 μm. Full size image In the lamprey, the parapineal organ forms a second pineal outgrowth at the midline, rostrally to the pineal organ [18] , [30] , and projects to the left habenulae, although this occurs at larval stages [33] ( Supplementary Fig. 3 ). Consistently, no evidence for parapineal evagination can be observed at stage 30 (that is, when L/R habenular identity is already visible), while the pineal stalk and evagination are clearly visible on sagittal sections ( Fig. 4r,s ). Importantly, the PmOtxB -expressing forebrain territory appears symmetric from stage 26 to 30 ( Fig. 4k–o ). The difference in size between the two habenulae observed from stage 27 thus does not correlate with overt asymmetry of the PmOtxB transcript distribution in the pineal field ( Fig. 4n–q ). Finally, analysis of neuronal projections in the catshark and lamprey embryonic brains through acetylated tubulin staining show no evidence of asymmetric fibres projecting from the pineal complex to the habenulae ( Fig. 4e–j,p,q ). Altogether, molecular characterizations provide no evidence of asymmetric cell migrations from the pineal primordium into the left habenulae at stages preceding, or concomitant with, the establishment of habenular asymmetry either in the catshark or the lamprey. Abrogation of nodal signalling leads to right isomerism The role of nodal signalling in the generation of epithalamic asymmetry can be directly analysed in the catshark and lamprey through pharmacological treatment using SB-505124. In the catshark, injection of the drug at stage 16, that is, immediately before the onset of nodal signalling activity in the diencephalon, leads 60–70 days later, at stage 31, to the following phenotype. Visceral organ asymmetry is maintained in these conditions, indicating that nodal activity later than stage 16 is not essential for visceral asymmetry establishment ( Supplementary Fig. 5a,b ). In contrast, habenular L/R asymmetry is lost in all SB-505124 injected embryos ( n =10; Fig. 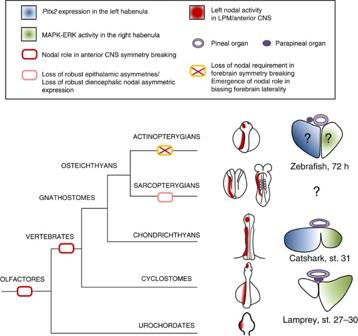Figure 6: Evolution of the role of nodal signalling in the formation of L/R asymmetries in the central nervous system. The evolutionary scenario shown is based on analyses conducted in representatives of olfactores (which include vertebrates and tunicates) and of the three major vertebrate taxa, that is, cyclostomes (or agnathans), chondrichthyans (or cartilaginous fishes) and osteichthyans (or bony fishes and tetrapods). Embryos at stages following neural tube closure are schematized to the right of the species tree in the zebrafish, xenopus/mouse, catshark, lamprey and in ciona, from top to bottom. Nodal expression in the LPM or in the diencephalon is shown in red. In line with its ancestrality in vertebrates, an asymmetric diencephalic expression has been observed in the lamprey, catshark and the zebrafish, but not in sarcopterygians thus far. Transverse sections of the developing epithalamus of actinopterygians, catshark and lamprey at the stages indicated are depicted on the right. The presence of pineal or parapineal organs (in light and dark purple, respectively) and their position relative to the habenulae are indicated. Whether the lamprey parapineal, which projects to the left habenula at larval stages, may contribute to the establishment of epithalamic asymmetries remains to be assessed, but our data suggest that it is not essential for initial symmetry breaking. A leftPitx2expression persisting in the habenulae when morphologically individualized (as observed in metamorphic flounder larvae16or the catshark, but not in the lamprey) is shown in blue and a right MAPK-ERK activity (as observed in the catshark and the lamprey) is shown in green. Conservation of right P-ERK and latePitx2expressions in the zebrafish remains to be assessed, as indicated by question marks. Boxes on the actinopterygian and sarcopterygian branches of the tree refer to diversifications of the role of nodal in the establishment of epithalamic diversifications in these lineages, the red box on the vertebrate branch refers to the ancestral role of nodal in symmetry breaking in the taxon, as inferred from comparisons between the catshark and lamprey. This role has also been reported in the anterior central nervous system ofC. intestinalis, suggesting its ancestrality in olfactores. 5 , Supplementary Table 6 ). First, in all treated embryos, the left habenulae decrease to a size comparable to their right counterpart, while a marked size difference in the anterior part of the organ is consistently observed at this stage in control and untreated embryos (compare Fig. 5a,b , Fig. 5c,d ). Second, all molecular markers tested become symmetrically expressed after treatment, with a right isomerism ( Supplementary Table 7 ). The left-sided ScPitx2 expression is completely lost ( Fig. 5a,b ), while the left and right catshark habenulae show a symmetric, right-sided like expression pattern of ScKctd12b (compare Fig. 5c,d ), ScKctd12a and ScKctd8 ( Supplementary Fig. 5c ). In particular, the specific left ScKctd12b -expressing territory normally observed in untreated or control embryos is undetectable in treated embryos ( Fig. 5c,d ). P-ERK expression, restricted to the right habenula in a control embryo as in all untreated embryos analysed, also becomes bilateral after treatment (compare Fig. 5e,f ). In contrast, the pineal rudiment appears appropriately specified, as assessed by its morphology and ScOtx5 expression in treated embryos ( Supplementary Fig. 5d,e ), making it unlikely that right habenular isomerism might be a secondary effect of pineal malformation. In the lamprey, SB-505124 treatments conducted from stages 21 to 24 also result in habenular defects at stages 27 and 30 ( Supplementary Tables 6 and 7 ). Similarly to treated catshark embryos, habenulae from treated lamprey embryos are completely symmetric, both in terms of size, which increases on the left to the size of the right habenula (compare Fig. 5g,i and Fig. 5h,j ), and of expression of P-ERK, which is expressed in both the right and left habenulae at stage 30, contrary to wild-type embryos (compare Fig. 5k and Fig. 5l ). In summary, based on size and molecular marker analysis, nodal abrogation leads to a right isomerism in the lamprey and the catshark developing epithalamus. Figure 5: Nodal abrogation induces a right isomerism in the catshark and lamprey epithalami. ( a – f ) Effect of SB-505124 treatment on habenular development in the catshark S. canicula . ( a – f ) Show transverse sections of stage 31 control embryos ( a , c , e ) and SB-505124-treated embryos ( b , d , f ), following hybridization with ScPitx2 ( a , b ) and ScKctd12b ( c , d ) probes, or following immunohistochemistry using an antibody directed against P-ERK ( e , f ). In ( a – d ), successive section planes are shown from anterior to posterior levels, with the same orientation as depicted in Fig. 2 . ( e , f ) Show sections at a median level. Red arrowheads in ( a , c ) point to left-sided hybridization signals present in control embryos but lost in SB-505124 treated embryos. White arrowheads in ( e ) point to P-ERK signals, restricted to the right in untreated or DMSO-injected embryos but found on both sides in SB-505124-treated embryos ( f ). A size difference is observed between the left and the right habenulae at anterior levels (larger on the left) in control embryos. Treated embryos exhibit a size reduction of the left habenula. ( g – l ) Effect of SB-505124 treatment on habenular development in the lamprey L. planeri . ( g – l ) Show transverse sections of stage 27 ( g , h ) and stage 30 ( k , l ) embryos following DAPI staining (blue) and immuno-histochemistry with an anti-acetylated tubulin ( g , h ; green) and an anti-P-ERK antibody ( k , l ; red). ( i ) and ( j ) show DAPI staining of the region boxed in ( g ) and ( h ), respectively, at higher magnification. Control embryos ( g , i , k ) exhibit a larger size of the right habenula and an asymmetric right P-ERK activity ( k ). In SB-505124-treated embryos ( h , j , l ), a size increase of the left habenula, resulting in a right isomerism, is observed ( j ) and the P-ERK signal is equally distributed between the left and right habenulae ( l ). Insets in ( k , l ) represent close-up views of the developing epithalamus. ( m ) Scheme showing molecular changes in habenulae of control and SB-505124-treated embryos. hc=habenular commissure; H L =left habenula; H R =right habenula; pi=pineal stalk. Scale bars: ( a – f ), 200 μm; ( g , l ), 100 μm. Full size image Our work investigates the role of nodal signalling in establishing L/R epithalamus asymmetry in the catshark and lamprey, providing novel insights into the ancestral role of nodal signalling in the vertebrate forebrain. We thus reveal the conservation of diencephalic and habenular molecular asymmetry across the three major vertebrate taxa, cyclostomes, chondrichthyans and osteichthyans, supporting the hypothesis that stereotyped L/R asymmetry directionality in the brain was already present in early vertebrates. Importantly though, and contrary to what has been described in the zebrafish [10] , [11] , [34] , we show that establishment of habenular asymmetric identity in the catshark and lamprey occurs through a nodal-dependent mechanism, in the absence of overt asymmetric development of the pineal field. These data shed new light on both the origin and evolution of the mechanisms controlling epithalamic asymmetries in vertebrates. From a mechanistic standpoint, nodal signalling appears as a conserved determinant of habenular L/R molecular identity in the lamprey and catshark, as assessed by the expression of L/R molecular markers. However, it differentially controls left habenulae size between the two species (its loss resulting in an increase in the lamprey and a reduction in the catshark). Conservation of molecular laterality between the two species indicates that relative habenulae size (larger on the left in the catshark but right in the lamprey) is not, in actual fact, a reliable indicator of L/R identity. This uncoupling may be related to different cellular roles of Nodal signalling in the catshark and the lamprey. An alternative hypothesis may be that nodal differentially controls the size of distinct habenular sub-territories occupying different proportions of the habenulae depending on species. Indeed, reiterated reciprocal expansions/contractions of conserved habenular subregions are known to have taken place during osteichthyan evolution [3] , [35] . Further analyses of the roles of nodal in the control of cell proliferation, apoptosis and neurogenesis, a process known to be essential to the generation of epithalamic asymmetries in the zebrafish [36] , [37] , should help to clarify this point. From an evolutionary standpoint, conservation of the role of nodal signalling in breaking habenular symmetry in both the catshark and lamprey suggests that it is likely to be an ancestral characteristic of vertebrates. Interestingly, this role appears largely lost in the zebrafish, as nodal abrogation results in a laterality shift rather than a loss of habenular asymmetries. However, in this species, nodal has also been shown to control an early asymmetric neurogenesis, preceding, and therefore independent of lateralized parapineal migration [37] . We propose that this role may be a vestigial heritage of an ancestral, parapineal independent nodal role, prevailing in early vertebrates and maintained in the lamprey and catshark ( Fig. 6 ). In support of this hypothesis, a role of nodal signalling in breaking symmetry has been previously reported in non-vertebrate deuterostomes and in protostomes, likely reflecting an ancient function of the pathway. Nodal abrogation thus induces a morphological symmetry of the sensory vesicle in ascidia [38] , the formation of an additional rudiment on the right side of the sea urchin larva [39] and a straight-shelled phenotype in gastropods [40] . Work in Ciona intestinalis [38] suggests that this ancestral function of nodal signalling may already have been operating in the anterior nervous system of olfactores, that is, before the emergence of vertebrates. Figure 6: Evolution of the role of nodal signalling in the formation of L/R asymmetries in the central nervous system. The evolutionary scenario shown is based on analyses conducted in representatives of olfactores (which include vertebrates and tunicates) and of the three major vertebrate taxa, that is, cyclostomes (or agnathans), chondrichthyans (or cartilaginous fishes) and osteichthyans (or bony fishes and tetrapods). Embryos at stages following neural tube closure are schematized to the right of the species tree in the zebrafish, xenopus/mouse, catshark, lamprey and in ciona, from top to bottom. Nodal expression in the LPM or in the diencephalon is shown in red. In line with its ancestrality in vertebrates, an asymmetric diencephalic expression has been observed in the lamprey, catshark and the zebrafish, but not in sarcopterygians thus far. Transverse sections of the developing epithalamus of actinopterygians, catshark and lamprey at the stages indicated are depicted on the right. The presence of pineal or parapineal organs (in light and dark purple, respectively) and their position relative to the habenulae are indicated. Whether the lamprey parapineal, which projects to the left habenula at larval stages, may contribute to the establishment of epithalamic asymmetries remains to be assessed, but our data suggest that it is not essential for initial symmetry breaking. A left Pitx2 expression persisting in the habenulae when morphologically individualized (as observed in metamorphic flounder larvae [16] or the catshark, but not in the lamprey) is shown in blue and a right MAPK-ERK activity (as observed in the catshark and the lamprey) is shown in green. Conservation of right P-ERK and late Pitx2 expressions in the zebrafish remains to be assessed, as indicated by question marks. Boxes on the actinopterygian and sarcopterygian branches of the tree refer to diversifications of the role of nodal in the establishment of epithalamic diversifications in these lineages, the red box on the vertebrate branch refers to the ancestral role of nodal in symmetry breaking in the taxon, as inferred from comparisons between the catshark and lamprey. This role has also been reported in the anterior central nervous system of C. intestinalis , suggesting its ancestrality in olfactores. Full size image This ancestral role of nodal is not exclusive of additional parapineal-dependent symmetry breaking mechanisms. The presence or absence of a parapineal organ appears as a highly variable trait across vertebrates and mechanisms responsible for this variability remain totally unknown. Interestingly, Pitx2 has recently been shown to be involved in restricting parapineal cell number in the zebrafish [41] . Thus, it is tempting to speculate that modulations of Pitx2 gene expression duration could account for parapineal variability. In line with this hypothesis, we report a correlation between the time-frame of Pitx2 expression in the catshark ( ScPitx2 persistent) and the lamprey ( PmPitxA restricted to a narrow developmental time window) and the absence (catshark) or presence (lamprey) of a parapineal organ. The key role of this organ in zebrafish suggests that its reiterated rise or regression across vertebrates may be a factor contributing to the diversification of habenular asymmetries. In teleosts, nodal signalling may thus have been recruited to bias laterality, possibly concomitantly with the emergence of a new parapineal-dependent mechanism, which now prevails in zebrafish ( Fig. 6 ). Whether additional habenular asymmetries may similarly be induced in a later phase in the lamprey, concomitantly with parapineal organ formation or differentiation, remains to be assessed. In conclusion, our data support the hypothesis that before the split between chondrichthyans and cyclostomes, nodal signalling provided a robust genetic mechanism underpinning symmetry breaking in the vertebrate forebrain, which then mostly evolved into a laterality overseer as observed in teleosts. Understanding whether, as in zebrafish [7] , [8] , habenular asymmetries controlled by this ancestral heritable mechanism may influence the processing and integration of sensory information in cyclostomes and chondrichthyans could reveal ancient adaptive mechanisms responsible for the fixation of this trait in the last common ancestor of vertebrates. Obtaining catshark and lamprey embryos Scyliorhinus canicula embryos were obtained from the Roscoff Marine Station and staged according to a selection of morphological criteria reported in refs 42 , 43 . Adult P. marinus were caught in April 2012 in Châteaulin (Brittany, France) and in June 2013 in Ulla River (northwestern Spain) during their upstream migratory phase and maintained in the laboratory at 17 °C in filtered fresh water until sexual maturation. Gametes were collected by gentle stripping and fertilized. Lampetra planeri embryos and larvae were provided by Guillaume Evanno (INRA, UMR 985 ESE, Rennes France). Lamprey embryos and prolarvae were raised in the laboratory in oxygenated fresh water at 17 °C. They were staged according to ref. 44 . All experiments were approved by the local ethic committee (Comité Rennais d'Ethique en matière d'Expérimentation Animale, C2EA-07, authorization n°R-2012-EG-02). Whole-mount in situ hybridization and sectioning ScNodal , ScVg1 , ScOtx5 and ScFgf8 antisense RNA probes were synthesized from cDNA fragments subcloned in pSPORT1 ( ScNoda l, ScVg1 and ScFgf8 ) or pTZ19R ( ScOtx5 ), and sequenced using Universal M13 primers as previously described [31] , [43] , [45] . GenBank accession codes for the corresponding sequences are KP698591 for ScNodal , KP698592 for ScVg1 , AAK85128.1 for ScOtx5 , KP698593 for ScFgf8 . The P. marinus PmOtxB probe was obtained by degenerate RT-PCR starting from stage 24 to 28 prolarval cDNAs, cloned into the pTZ19U vector and characterized by sequencing using the universal primers M13_pUC_rev and M13_pUC_fwd. ScPitx2 , ScKctd12a , ScKctd12b, ScLeftyB and PmLefty probes were obtained from collections of embryonic S. canicula or prolarval P. marinus cDNA recombinants, characterized by Sanger sequencing and described in refs 43 , 46 . Cloning of the ScGfi1 , ScKctd8 and PmKctd12 gene fragment and riboprobe synthesis are described in Supplementary Table 4 . Genbank accession codes for the corresponding sequences are shown in Supplementary Table 1 . Blast searches in the current P. marinus genome failed to identify a Gfi1 orthologue. Clone identities were confirmed by the phylogenetic analyses presented in Supplementary Fig. 1 . For in situ hybridizations, digoxigenin-labelled antisense RNA probes were prepared from the selected clones. Whole-mount and section in situ hybridizations were conducted using standard protocols adapted to the catshark and lamprey as previously described [43] , [47] , [48] . All P. marinus probes showed strong hybridization signals in hybridizations of L. planeri prolarvae, with indistinguishable expression characteristics. Immunohistochemistry on lamprey and catshark sections Specimens fixed in 4% PFA were rinsed in 1 × PBS, dehydrated, embedded in paraffin and cut on a microtome (Leica, 10–12 μm thick). After epitope unmasking, sections were subjected to immunohistochemistry with an anti-P-ERK (Sigma M-8159, 1:2,000) or an anti-acetylated tubulin (Sigma T-6793, 1:1,000) antibody, using the TSA Plus System kit (Perkin Elmer) according to the manufacturer’s conditions. Nuclear staining was achieved using DAPI or YOYO-3 dye (Invitrogen). Representative embryo sections were scanned with a Leica SP5 confocal laser-scanning microscope. Pharmacological treatments of embryos with a nodal inhibitor Developing lamprey embryos or catshark embryos were treated with SB-505124 diluted in DMSO, an inhibitor of transforming growth factor-β type I receptors ALK4, ALK5 and ALK7 (ref. 49 ). For short duration treatments on catshark embryos, 200 μl of a solution containing 500 μM SB-505124 was injected into the egg case and through the shell either at stages 13 to 14, or at stages 15 to 16. In both cases, the eggs were maintained in oxygenated sea water at 17 °C for 3 days before embryo fixation. Viability in these conditions was higher than 90% in control and treated embryos, but treated embryos failed to survive until stage 31 (while no mortality was observed in control ones). To overcome these lethality problems, the same volume was injected per egg but the drug concentration was lowered to 50 μM for long-term treatments. In this case, the drug was injected at stages 15–16, and the eggs were incubated in oxygenated sea water at 17 °C for ~2 months, until embryos reached stage 31. The effect of the 50 μM drug concentration on ScPitx2 expression at stage 17–18 was also assessed following a 3-day incubation after injection ( Supplementary Table 3 ). In the lamprey, for short-duration treatments, developing embryos ( Petromyzon marinus and Lampetra planeri ) were placed from stage 21 to 24 into a culture plate containing fresh water with 25 or 75 μM SB-505124 ( Fig. 1 and Supplementary Table 3 ). Long-duration treatments were conducted in Lampetra planeri , using 25 and 50 μM SB-505124 concentrations. Developing embryos were incubated in the presence of the drug from stage 21 to 24 and in fresh water at subsequent stages. A massive mortality (>90%) was observed at stage 26 at the highest drug concentration used (50 μM SB-505124 concentration), and only embryos exposed to a 25 μM SB-505124 concentration were further maintained in culture until fixation at stages 27 and 30. The viability in the latter conditions was >90%. The effect of this concentration was also assessed on PmLefty expression at stage 24 ( Supplementary Table 3 ). Both in the catshark and lamprey, the same protocol was conducted in parallel for control embryos, except that the injected solution did not contain the drug. Accession codes : The sequences generated in this study have been deposited in GenBank nucleotide database under the accession codes KF190312 to KJ190316 , KM041048 , KM041049 , KJ623814 , KJ623815 . How to cite this article: Lagadec, R. et al . The ancestral role of nodal signalling in breaking L/R symmetry in the vertebrate forebrain. Nat. Commun. 6:6686 doi: 10.1038/ncomms7686 (2015).